Phytochrome and retrograde signalling pathways converge to antagonistically regulate a light-induced transcriptional network Plastid-to-nucleus retrograde signals emitted by dysfunctional chloroplasts impact photomorphogenic development, but the molecular link between retrograde- and photosensory-receptor signalling has remained unclear. Here, we show that the phytochrome and retrograde signalling (RS) pathways converge antagonistically to regulate the expression of the nuclear-encoded transcription factor GLK1, a key regulator of a light-induced transcriptional network central to photomorphogenesis. GLK1 gene transcription is directly repressed by PHYTOCHROME-INTERACTING FACTOR (PIF)-class bHLH transcription factors in darkness, but light-activated phytochrome reverses this activity, thereby inducing expression. Conversely, we show that retrograde signals repress this induction by a mechanism independent of PIF mediation. Collectively, our data indicate that light at moderate levels acts through the plant’s nuclear-localized sensory-photoreceptor system to induce appropriate photomorphogenic development, but at excessive levels, sensed through the separate plastid-localized RS system, acts to suppress such development, thus providing a mechanism for protection against photo-oxidative damage by minimizing the tissue exposure to deleterious radiation. Interorganellar communication coordinates gene expression of nuclear and organelle genomes and is essential to ensure cell fitness. In some eukaryotes, bidirectional communication between mitochondria and nucleus regulates the processes such as life span (yeast), cell cycle ( Drosophila ) or tumour progression (animal cells) [1] . In plants, where the majority of chloroplast components are encoded in the nucleus, anterograde regulation from nucleus to chloroplast and retrograde signalling (RS) from chloroplast to nucleus, are critical to adjust chloroplast biogenesis and photosystem assembly to the prevailing environment and chloroplast status [2] , [3] , [4] . Despite the important implications of RS on cellular function in all organisms, insight into the underlying mechanisms remains sparse. Deetiolation is the critical switch from skotomorphogenic to photomorphogenic development, triggered in the seedlings emerging from subterranean darkness into sunlight, and is characterized by an extensive transcriptional reprogramming that drives the morphological changes necessary to establish a normal green photosynthetically active seedling [5] . In the dark, skotomorphogenic seedlings use fast-growing hypocotyls to rapidly reach the soil surface, together with a protective apical hook and appressed cotyledons with undeveloped chloroplasts. In contrast, light inhibits hypocotyl elongation and stimulates cotyledon separation and expansion, congruent with the development of functional chloroplasts, thus enabling light capture for photosynthesis. A subgroup of basic helix-loop-helix transcriptional regulators, termed phytochrome-interacting factors(PIFs), accumulate in the dark and promote skotomorphogenesis through regulation of about 10% of the genes in the genome [6] . Light exposure activates the phytochrome family of red and far-red light-responsive photoreceptors that directly interact with the PIFs and trigger their proteolytic degradation, thereby redirecting gene expression to drive deetiolation [7] , [8] , [9] . Indicative of the central role of the PIFs in this process, a dark-grown quadruple pifq mutant, deficient in four PIFs (PIF1, PIF3, PIF4 and PIF5), largely phenocopies wild-type (WT) seedlings grown in the light at both the morphological and transcriptional levels. These mutant seedlings display a constitutively photomorphogenic ( cop -like) phenotype, which includes partially developed chloroplasts [10] , [11] . On the basis of the phenotypes of plants with induced plastid dysfunctionality, plastid signals have been reported to impact normal light-regulated development [12] , [13] , [14] , [15] . Although the evidence indicates that RS can repress some aspects of early seedling photomorphogenic development, in addition to affecting chloroplast biogenesis [12] , [13] , [14] , [15] , mechanistic insight into the connection between the photomorphogenic and RS pathways has been lacking. While many of the components of the phytochrome pathway (PIFs) and the RS pathway (GUN1, GLK1) examined in the present work have been reported in a number of publications [9] , [10] , [12] , [16] , [17] , [18] , here we present data that connect the two in a comprehensive fashion, identifying the molecular framework that integrates the two pathways at a central node at the apex of a transcriptional network that regulates early seedling photomorphogenic development. We show that the phytochrome and the GUN1 RS pathways act antagonistically to control the expression of GLK1 , a key transcriptional regulator of photomorphogenesis directly repressed by the PIFs in the dark. Whereas light at moderate levels acts through the phytochrome/PIF sensory-photoreceptor system to induce GLK1 expression and photomorphogenic development, light at excessive levels is sensed by the plastid and represses GLK1 induction and photomorphogenesis through a GUN1-mediated RS mechanism independent of PIF mediation. Our data indicate that RS provides a mechanism for protection against photo-oxidative damage by minimizing the tissue exposure to deleterious radiation. Retrograde signals suppress PIF-mediated photomorphogenesis As an experimental system, we treated light-grown seedlings with lincomycin, a drug known to activate RS by inhibiting chloroplast biogenesis [19] . Strikingly, we found that WT seedlings grown on lincomycin in white light resembled dark-grown seedlings, with long hypocotyls and appressed unexpanded cotyledons that did not accumulate chlorophyll ( Fig. 1a,b ). This effect was also observed under red light ( Supplementary Fig. 1 ) and after treatment with norflurazon, a herbicide that inhibits carotenoid biosynthesis and causes photo-oxidative damage of chloroplasts in white light [20] , [21] ( Supplementary Fig. 2 ). The effect of lincomycin on the early development of WT seedlings observed here was considerably stronger than in some previous studies [12] , [22] . This discrepancy may have resulted from these studies having used seedlings grown on 2% sucrose (which we did not administer in our experiments), or from differences in the light conditions. It is well-documented that exogenous sucrose significantly alters normal light-regulated gene-expression and metabolic-pathway patterns, together with associated deviations in growth and developmental responses [23] , [24] , [25] , [26] . On the other hand, our findings are similar to, and extend, other studies showing that defects in chloroplast biogenesis produced by mutations in the SIGMA 2 and 6 components of the chloroplast RNA polymerase (which induce RS similarly to lincomycin) [27] prevented normal seedling photomorphogenesis under continuous light ( Supplementary Fig. 3 ) [28] . When we examined the kinetics of the deetiolation process, we found that the rapid cotyledon separation response, normally exhibited by dark-grown WT seedlings upon light exposure, was nearly completely blocked in the presence of lincomycin, consistent with the end point analysis ( Fig. 1c ). We also observed an inhibitory effect on the rapid hook-opening response, indicating that lincomycin has an early effect on hook development. However, this recovered over time and is not detectable in the end point analysis. These observations suggest that RS activity either pre-exists or can be deployed very rapidly in defective plastids, to prevent the normal light-induced response in the seedling apex, very early during deetiolation. In addition, our results indicate that the effects of RS induced by defects in plastid function, are not confined to chloroplast biogenesis, but rather pleiotropically repress seedling photomorphogenesis in the light [15] . This conclusion raises the possibility that the informational-light-induced, PIF-mediated transcriptomic changes that normally implement the photomorphogenic programme, in response to activation of the sensory-photoreceptor pathways, might be affected under these conditions. A previous study showing significant overlap between the transcriptomic changes induced by lincomycin and by a shift from low-to-high fluence-rate white- or blue-light [14] supports this possibility. 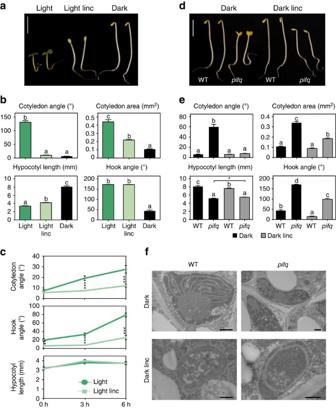Figure 1: RS from the chloroplast suppresses PIF-mediated seedling photomorphogenesis. (a) Lincomycin treatment preventsArabidopsisseedling deetiolation in continuous white light. WT seedlings were grown for 3 days in the light in the absence (Light) or presence (Light linc) of lincomycin. For comparison, 3-day-old dark-grown seedlings are shown at right. Scale bar, 2.5 mm. (b) Cotyledon angle and area, hypocotyl length and hook angle of seedlings grown as in a. (c) Lincomycin inhibits early deetiolation during the transition of dark-grown seedlings to light. Quantification of cotyledon angle (top), hook angle (middle) and hypocotyl length (bottom) of 2-day-old dark-grown WT seedlings transferred to white light for the indicated times, grown in the absence (dark green) or presence (light green) of lincomycin. (d) Lincomycin treatment suppresses thecop-like phenotype ofpifqseedlings in the dark. WT andpifqseedlings were grown for 3 days in the dark in the absence (Dark) or presence (Dark linc) of lincomycin. (e) Cotyledon angle and area, hypocotyl length and hook angle of seedlings grown as in d. (f) Higher-magnification micrographs of samples prepared as in d. Representative etioplasts are shown for WT (left) andpifq(right) seedlings grown in absence (top) or presence (bottom) of lincomycin. Scale bar, 500 nm. Error bars inb,canderepresent s.e.m. (n⩾20). The experiments were repeated two times with similar results. Inb,edifferent letters denote statistically significant differences among means by Tukey-b test (P<0.05). Incande, statistically significant differences between mean values by Student’st-test are shown (*P<0.05; **P<0.01 and ***P<0.001). Figure 1: RS from the chloroplast suppresses PIF-mediated seedling photomorphogenesis. ( a ) Lincomycin treatment prevents Arabidopsis seedling deetiolation in continuous white light. WT seedlings were grown for 3 days in the light in the absence (Light) or presence (Light linc) of lincomycin. For comparison, 3-day-old dark-grown seedlings are shown at right. Scale bar, 2.5 mm. ( b ) Cotyledon angle and area, hypocotyl length and hook angle of seedlings grown as in a. ( c ) Lincomycin inhibits early deetiolation during the transition of dark-grown seedlings to light. Quantification of cotyledon angle (top), hook angle (middle) and hypocotyl length (bottom) of 2-day-old dark-grown WT seedlings transferred to white light for the indicated times, grown in the absence (dark green) or presence (light green) of lincomycin. ( d ) Lincomycin treatment suppresses the cop -like phenotype of pifq seedlings in the dark. WT and pifq seedlings were grown for 3 days in the dark in the absence (Dark) or presence (Dark linc) of lincomycin. ( e ) Cotyledon angle and area, hypocotyl length and hook angle of seedlings grown as in d. ( f ) Higher-magnification micrographs of samples prepared as in d. Representative etioplasts are shown for WT (left) and pifq (right) seedlings grown in absence (top) or presence (bottom) of lincomycin. Scale bar, 500 nm. Error bars in b , c and e represent s.e.m. ( n ⩾ 20). The experiments were repeated two times with similar results. In b , e different letters denote statistically significant differences among means by Tukey-b test ( P <0.05). In c and e , statistically significant differences between mean values by Student’s t -test are shown (* P <0.05; ** P <0.01 and *** P <0.001). Full size image To examine this potential PIF involvement genetically, we analysed pifq mutants in the presence of lincomycin. We reasoned that if the PIF-regulated network is also targeted by RS to inhibit photomorphogenesis in the light, we should detect an effect on the photomorphogenic phenotype induced by the absence of the PIF-quartet in the pifq mutant in the dark. Strikingly, we found that lincomycin does indeed strongly suppress the cop -like phenotype of pifq in the dark ( Fig. 1d,e ; Supplementary Fig. 4 ). The drug completely suppressed cotyledon separation in pifq seedlings, sustained hook curvature, and restored cotyledon appression to levels similar to those exhibited by etiolated WT seedlings in darkness. Lincomycin also induced a modest (1 mm) but statistically significant (Student’s t -test) increase in hypocotyl elongation in pifq seedlings compared with the untreated control (see Fig. 1d,e ; Supplementary Fig. 4 ). Partial suppression of the constitutive photomorphogenic phenotype was also observed in dark-grown cop1 seedlings in the presence of lincomycin ( Supplementary Fig. 5 ), in agreement with the notion that the constitutively photomorphogenic phenotype of cop1 in the dark might be caused, in part, by the lower accumulation of PIFs seen in cop1 (ref. 29 ), and consistent with previous results in pea [19] . In contrast to lincomycin, norflurazon treatment did not induce RS and did not affect the phenotype of pifq in the dark ( Supplementary Fig. 6 ), in agreement with the fact that light is needed to induce RS in carotenoid-deficient seedlings [20] , [21] . In dark-grown WT seedlings, lincomycin did not alter the etiolated phenotype, having only a minor effect on hook curvature ( Fig. 1d,e ; Supplementary Fig. 4 ). At the subcellular level, treatment with lincomycin interfered with plastid development in both WT and pifq dark-grown seedlings, preventing the partial differentiation of etioplasts into chloroplasts observed in non-treated pifq seedlings in the dark ( Fig. 1f ). RS antagonize the light induction of PIF-repressed genes Because defects in chloroplast biogenesis activate RS, and activation of RS is well-known to regulate nuclear gene expression [14] , [23] , we analysed whether RS might indeed be able to target the PIF-regulated transcriptome during early seedling development. For this purpose, we initially used published data [11] , [23] , [27] . Interestingly, of 871 previously defined red light-induced genes [11] , 457 (52%) are inhibited in their normal light responsiveness by RS (in agreement with Ruckle et al . [14] ), and of those, 343 (75%) correspond to genes shown previously [11] to be repressed by the PIFs in the dark ( Fig. 2a ; Supplementary Data 1 ). We labelled these 343 genes as ‘Gene-Set PIF-RS’ (for PIF- and RS-repressed). Moreover, the expression levels of this gene-set in WT seedlings grown in the presence of light and lincomycin resembled those in untreated WT in the dark, indicating that RS is, directly or indirectly, blocking their light responsiveness ( Fig. 2b ; Supplementary Fig. 7 ). Importantly, our analysis shows further that this congruent regulation of gene expression by RS and PIFs is strongly selective for light-induced/PIF-repressed genes, because only 19 of the 313 previously identified light-repressed/PIF-induced genes [11] were re-induced by lincomycin in light-grown WT seedlings, and their expression level was not restored to WT-dark levels ( Supplementary Fig. 8 ). These results suggest that RS inhibits deetiolation, at least partly, by antagonizing the light-induced expression of a large set of PIF-repressed genes, without altering the normal light-triggered repression of the PIF-induced gene set. 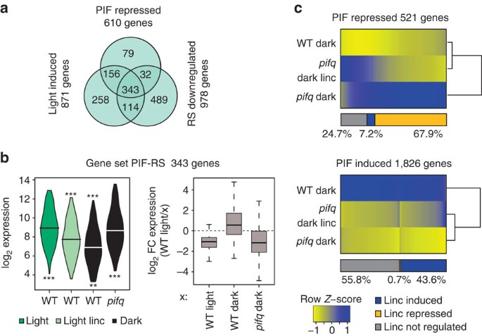Figure 2: Retrograde signals repress the light-induced expression of PIF-repressed genes. (a) Plastid signals repress the induction of light-induced genes. Overlap among genes downregulated by chloroplast RS27, induced by red-light11or repressed by PIFs in the dark11, identifies 343 genes labelled as ‘Gene-Set PIF-RS’ (gene lists provided inSupplementary Data 1). (b) Expression of genes in ‘Gene-Set PIF-RS’ in WT andpifqmutants grown in the light in the absence (dark green) or presence (light green) of lincomycin, or in the dark (black) (left). Fold-change expression of genes in ‘Gene-Set PIF-RS’ between WT light lincomycin with respect to WT light, WT dark orpifqdark (right). Data obtained from refs11and23. Statistically significant differences from WT light or WT light linc by heteroscedastict-test are indicated in the upper and lower part, respectively (**P<0.01 and ***P<0.001). (c) Lincomycin extensively restores the PIF-repressed network inpifqin the dark to the WT levels. Two-dimensional-cluster diagram depicting expression levels of 521 PIF-repressed (top) and 1,826 PIF-induced (bottom) SSTF genes in the dark in the absence (dark) or presence (dark linc) of lincomycin. Genes were identified by transcriptomic profiling of seedlings grown for 3 days in the dark in the absence (dark) or presence (dark linc) of lincomycin. Figure 2: Retrograde signals repress the light-induced expression of PIF-repressed genes. ( a ) Plastid signals repress the induction of light-induced genes. Overlap among genes downregulated by chloroplast RS [27] , induced by red-light [11] or repressed by PIFs in the dark [11] , identifies 343 genes labelled as ‘Gene-Set PIF-RS’ (gene lists provided in Supplementary Data 1 ). ( b ) Expression of genes in ‘Gene-Set PIF-RS’ in WT and pifq mutants grown in the light in the absence (dark green) or presence (light green) of lincomycin, or in the dark (black) (left). Fold-change expression of genes in ‘Gene-Set PIF-RS’ between WT light lincomycin with respect to WT light, WT dark or pifq dark (right). Data obtained from refs 11 and 23 . Statistically significant differences from WT light or WT light linc by heteroscedastic t -test are indicated in the upper and lower part, respectively (** P <0.01 and *** P <0.001). ( c ) Lincomycin extensively restores the PIF-repressed network in pifq in the dark to the WT levels. Two-dimensional-cluster diagram depicting expression levels of 521 PIF-repressed (top) and 1,826 PIF-induced (bottom) SSTF genes in the dark in the absence (dark) or presence (dark linc) of lincomycin. Genes were identified by transcriptomic profiling of seedlings grown for 3 days in the dark in the absence (dark) or presence (dark linc) of lincomycin. Full size image Newly performed RNA-seq-based transcriptomic analysis here of dark-grown, non-drug-treated, WT and pifq seedlings, identified 521 PIF-repressed and 1,826 PIF-induced genes whose expression changed statistically significantly and by at least twofold (SSTF) in 3-day-old pifq seedlings compared with WT in the absence of light (see Supplementary Note 1 for a detailed description of the analysis). Lincomycin strongly, but selectively, reversed this pifq molecular phenotype, extensively and preferentially restoring the status of the PIF-repressed network in the pifq mutant to WT levels ( Fig. 2c ; Supplementary Note 1 ), by statistically significantly repressing the expression of 68% (354) of the PIF-repressed SSTF genes ( Supplementary Figs 9 and 10 ; Supplementary Note 1 ; Supplementary Data 2 ). This 354-gene set corresponds predominantly to PIF-repressed/light-induced genes that have been shown in previous reports to be downregulated by RS in the light in WT seedlings [27] , and largely overlaps with the ‘Gene-Set PIF-RS’ defined above ( Supplementary Note 1 ; Supplementary Fig. 11 ). Interestingly, only 9–13% of the genes in these sets are direct PIF targets ( Supplementary Fig. 12 ) [16] , suggesting indirect regulation of the majority by the PIFs. The two largest represented groups correspond to chloroplast- and nuclear-localized proteins ( Supplementary Fig. 13 ). These results show that activation of RS in the dark reverses the expression of the transcriptional network induced in pifq , concomitant with the suppression of the cop -like seedling phenotype of the mutant. Altogether, our findings indicate that the RS preferentially targets the PIF-repressed genes in restraining light-induced deetiolation. This conclusion is in contrast to a previous model proposing the converse, namely, that integration of the RS and photoreceptor-mediated light signals was accomplished via informational-light induction of genes that were further induced by the RS [14] . Moreover, our findings suggest that the RS and informational-light-regulated signalling pathways must converge downstream of the PIFs to antagonistically regulate the initiation of seedling photomorphogenesis. This conclusion is in contrast to a previous model based on small differences detected in hy5 mutants, proposing that the RS ‘rewires’ the light signalling network in a manner that converts informational light from a positive to a negative signal and vice versa, through transforming HY5 from a positive to a negative regulator of gene expression [13] . Our findings support a model for PIF-regulated genes, in which RS represses the light induction of PIF-repressed genes by a mechanism that acts in the absence of the PIF proteins and, therefore, is independent of any direct RS regulation of PIF transcriptional activity. GUN1-mediated RS antagonizes PIF-regulated gene expression To begin to gain further insight into how the RS pathway might converge on the PIF-regulated transcriptional network, we treated light-grown abi4 , gun1 , gun5 and gun6 mutant seedlings with lincomycin. GUN1 and ABI4 are two major described mediators of the RS pathway [23] , and GUN5 and GUN6 are involved in plastid-to-nucleus signal transduction [21] , [30] . We found that lincomycin prevented full deetiolation of abi4 , gun5 , and gun6 seedlings in the light, similarly to WT ( Fig. 3a,b ; Supplementary Figs 14 and 15 ). However, in striking contrast, gun1 seedlings partially deetiolated in the presence of lincomycin in the light, displaying light-imposed inhibition of hypocotyl elongation and open and expanded cotyledons ( Fig. 3a,b ; Supplementary Figs 14 and 15 ). To examine the molecular phenotypes, we assessed the role of GUN1 and ABI4 in the regulation of the expression of the ‘Gene-Set PIF-RS’ defined above. By analysing the available expression data for gun1 and abi4 (ref. 23 ), we found that these genes responded strongly to lincomycin in WT and abi4 , but not in gun1 , which displayed gene expression levels in lincomycin-grown seedlings, comparable to those of seedlings not treated with lincomycin ( Fig. 3c,d ). From these collective data, we conclude that GUN1, but likely not ABI4, GUN5 or GUN6, is necessary for the production, transmission or implementation of the lincomycin-induced RS that inhibits the photoreceptor-mediated, light-induced expression of a subset of light-induced/PIF-repressed genes, thereby repressing seedling photomorphogenesis in the light in response to chloroplast dysfunction. 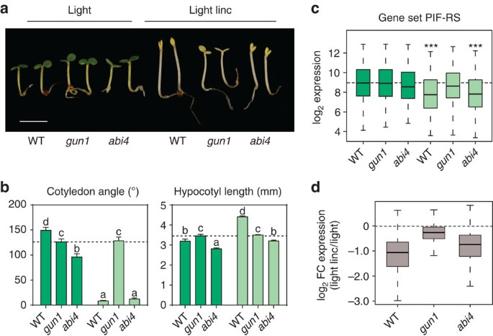Figure 3: GUN1 mediates the RS that antagonizes PIF-regulated gene expression. (a) Mutants inGUN1partially deetiolate in the light in the presence of lincomycin, whereas response of mutants inABI4responded more similar to WT. WT,abi4andgun1seedlings were grown for 3 days in white light in the absence (Light) or presence (Light linc) of lincomycin. Scale bar, 2.5mm. (b) Cotyledon angle and hypocotyl length of seedlings grown as in a. Error bars represent the s.e.m. of two independent experiments, each time sampling (n⩾25). Different letters denote statistically significant differences among means by Tukey-b test (P<0.05). (c) Lincomycin-induced repression in gene expression in the light of the 343 genes in ‘Gene-Set PIF-RS’ is blocked ingun1. Expression of genes in ‘Gene-Set PIF-RS’ in WT,abi4andgun1in the absence (dark green) and presence (light green) of lincomycin. Statistically significant differences from WT light by heteroscedastict-test are indicated (***P<0.001). (d) Fold-change expression in the light in the presence (Light linc) with respect to absence (Light) of lincomycin in WT,abi4andgun1seedlings. Data forc,dwere obtained from ref.23. Figure 3: GUN1 mediates the RS that antagonizes PIF-regulated gene expression. ( a ) Mutants in GUN1 partially deetiolate in the light in the presence of lincomycin, whereas response of mutants in ABI4 responded more similar to WT. WT, abi4 and gun1 seedlings were grown for 3 days in white light in the absence (Light) or presence (Light linc) of lincomycin. Scale bar, 2.5mm. ( b ) Cotyledon angle and hypocotyl length of seedlings grown as in a. Error bars represent the s.e.m. of two independent experiments, each time sampling ( n ⩾ 25). Different letters denote statistically significant differences among means by Tukey-b test ( P <0.05). ( c ) Lincomycin-induced repression in gene expression in the light of the 343 genes in ‘Gene-Set PIF-RS’ is blocked in gun1 . Expression of genes in ‘Gene-Set PIF-RS’ in WT, abi4 and gun1 in the absence (dark green) and presence (light green) of lincomycin. Statistically significant differences from WT light by heteroscedastic t -test are indicated (*** P <0.001). ( d ) Fold-change expression in the light in the presence (Light linc) with respect to absence (Light) of lincomycin in WT, abi4 and gun1 seedlings. Data for c , d were obtained from ref. 23 . Full size image PIFs and RS antagonistically regulate GLK1 transcription Because the GUN1 gene does not appear to bind PIFs in its promoter [16] , and is not a PIF-regulated gene ( Supplementary Data 2 ), phytochrome-mediated light- and plastid-RS signalling must converge downstream of both GUN1 and the PIFs, likely through co-regulation of one or more common target genes. Interestingly, analysis of DNA-binding motifs revealed that the ‘Gene-Set PIF-RS’ is significantly and specifically enriched in the putative GLK-binding site CCAATC ( z -score=5.35; Fig. 4a ) [17] . GLK1 is a PIF-repressed gene, which is directly targeted by PIFs in the dark [16] , [31] , [32] ( Supplementary Fig. 16 ), and that has been proposed to respond to RS downstream of GUN1 (refs 17 and 18 ). This evidence suggested to us that GLK1 might provide clues to the link between informational-light/PIF and RS/GUN1 signalling. Consistent with this notion, GLK1 expression is induced in light-grown WT seedlings, as well as being upregulated in pifq in the dark [11] , [16] . We found also that the expression induced in both conditions was largely suppressed by lincomycin, and in a GUN1-dependent fashion (at least in the light) extending previous findings [17] ( Fig. 4b ). These results indicate that RS acts on or upstream of GLK1 . Moreover, a similar expression pattern was observed for a set of 93 genes previously defined as GLK1-induced [17] ( Fig. 4c ). In addition, the PIF-RS gene set is enriched in GLK1 -regulated genes, and GLK1 -bound genes are enriched in PIF-RS genes ( Supplementary Fig. 17 ). Taken altogether, these results indicate that GLK1 is transcriptionally targeted, in antagonist fashion, by informational-light and GUN1-facilitated-retrograde signals, which induce and repress GLK1 expression, respectively, to regulate a subset of PIF-RS-controlled genes. Our results also indicate that GLK1 is not regulated under these conditions by either ABI4 ( Supplementary Fig. 18 ; in agreement with our findings presented in Fig. 3c,d ) or by HY5, which was previously proposed to respond to RS [13] ( Supplementary Fig. 19 ). 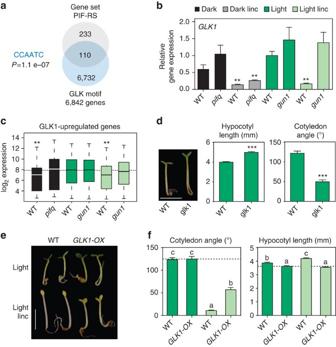Figure 4: Retrograde and PIF-mediated light signals antagonistically regulate deetiolation through transcriptional control ofGLK1. (a) Promoter regions (500 bp upstream of the start codon) of PIF-RS genes are significantly enriched in putative GLK-binding motifs (CCAATC)17, present in 6,842 promoter regions in theArabidopsisgenome. (b)GLK1is a gene whose expression is repressed by the PIFs in the dark and by lincomycin in a GUN1-dependent fashion in the light. Transcript levels ofGLK1analysed by qRT–PCR in 3-day-old WT,pifqandgun1seedlings grown in the dark or in continuous white light in the absence (Dark and Light, respectively) or presence (Dark linc and Light linc, respectively) of lincomycin. Values were normalized toPP2A, and expression levels are expressed relative to WT light set at one. Data are the means±s.e.m. of biological triplicates (n=3). (c) GLK1-induced genes display a pattern of expression similar toGLK1. Transcript levels were obtained from refs11and23, for a set of 93 genes previously defined as GLK1-induced17, which are represented in the ATH1 array. Statistically significant differences from WT Light by heteroscedastict-test are indicated (**P<0.01). (d) GLK1 promotes photomorphogenesis under continuous white light. WT andglk1mutant seedlings grown for 3 days in the light display a hyposensitive phenotype with partially closed cotyledons and longer hypocotyls. Scale bar, 2.5 mm. (e) Seedlings overexpressingGLK1display insensitivity to lincomycin and partially deetiolate in the presence of lincomycin. WT andGLK1-OXseedlings were grown for 3 days in white light in the absence (Light) or presence (Light linc) of lincomycin. Scale bar, 2.5 mm. (f) Cotyledon angle and hypocotyl length of seedlings grown as in e. Letters denote the statistically significant differences among means by Tukey-b test (P<0.05). Error bars ind,frepresent s.e.m. of two independent experiments (n⩾20). Inbandd, statistically significant differences from light-grown WT seedlings by Student’st-test are shown (**P<0.01 and ***P<0.001). Figure 4: Retrograde and PIF-mediated light signals antagonistically regulate deetiolation through transcriptional control of GLK1 . ( a ) Promoter regions (500 bp upstream of the start codon) of PIF-RS genes are significantly enriched in putative GLK-binding motifs (CCAATC) [17] , present in 6,842 promoter regions in the Arabidopsis genome. ( b ) GLK1 is a gene whose expression is repressed by the PIFs in the dark and by lincomycin in a GUN1-dependent fashion in the light. Transcript levels of GLK1 analysed by qRT–PCR in 3-day-old WT, pifq and gun1 seedlings grown in the dark or in continuous white light in the absence (Dark and Light, respectively) or presence (Dark linc and Light linc, respectively) of lincomycin. Values were normalized to PP2A , and expression levels are expressed relative to WT light set at one. Data are the means±s.e.m. of biological triplicates ( n =3). ( c ) GLK1-induced genes display a pattern of expression similar to GLK1 . Transcript levels were obtained from refs 11 and 23 , for a set of 93 genes previously defined as GLK1-induced [17] , which are represented in the ATH1 array. Statistically significant differences from WT Light by heteroscedastic t -test are indicated (** P <0.01). ( d ) GLK1 promotes photomorphogenesis under continuous white light. WT and glk1 mutant seedlings grown for 3 days in the light display a hyposensitive phenotype with partially closed cotyledons and longer hypocotyls. Scale bar, 2.5 mm. ( e ) Seedlings overexpressing GLK1 display insensitivity to lincomycin and partially deetiolate in the presence of lincomycin. WT and GLK1-OX seedlings were grown for 3 days in white light in the absence (Light) or presence (Light linc) of lincomycin. Scale bar, 2.5 mm. ( f ) Cotyledon angle and hypocotyl length of seedlings grown as in e. Letters denote the statistically significant differences among means by Tukey-b test ( P <0.05). Error bars in d , f represent s.e.m. of two independent experiments ( n ⩾ 20). In b and d , statistically significant differences from light-grown WT seedlings by Student’s t -test are shown (** P <0.01 and *** P <0.001). Full size image To test whether the transcriptional regulation of GLK1 by light and RS might be relevant to seedling photomorphogenesis, we examined the phenotype of seedlings with altered GLK1 expression. We reasoned that if GLK1 is a key link regulating photomorphogenesis downstream of both sensory-photoreceptor-mediated light signalling and RS, glk1 mutants should exhibit alterations in response to activation of these pathways. In agreement with this proposal, glk1 seedlings were indistinguishable from the WT in the dark but displayed longer hypocotyls and less separated cotyledons when grown in the light ( Fig. 4d ; Supplementary Fig. 20 ), indicating that GLK1 acts positively in seedling photomorphogenic development. Seedlings constitutively expressing GLK1 under the control of the 35 S promoter ( GLK1-OX ), were similar to WT in the dark although did show slightly shorter hypocotyls ( Supplementary Fig. 20b ), but, in striking contrast to WT, partially deetiolated in the presence of lincomycin in response to light, as indicated by short hypocotyls, and open and expanded cotyledons ( Fig. 4e,f ), and displayed high LHCB expression in lincomycin-treated seedlings, similarly to gun1 ( Supplementary Fig. 21 ). In contrast to GLK1 , the closely related GLK2 gene appears to have a minor role in this process ( Supplementary Fig. 22 ). These findings extend and refine the previously described role of GLK1 as a regulator of photosynthetic-apparatus-gene expression [17] , to define it as a previously unrecognized positive factor that acts pleiotropically to orchestrate the broader photomorphogenic programme. Altogether with the evidence that GLK1 is a direct target of PIF-imposed repression, the data support the conclusion that GLK1 is a pivotal target directly at the convergence of the informational-light/PIF and RS/GUN1 signalling pathways. This conclusion implies strongly in turn, that the GUN1-facilitated, RS-imposed repression of the light-induced expression of GLK1 , that is otherwise necessary for deetiolation, provides a mechanism to attenuate seedling photomorphogenesis in the event of chloroplast disruption. Such disruption has been shown to activate RS under natural environments triggered by excess light [33] , [34] , highlighting the likely biological significance of this proposed attenuation mechanism. High-intensity light inhibits PIF-mediated deetiolation To investigate the proposed mechanism and the role of PIF-RS-regulated GLK1 expression more closely, we examined the consequences of exposing dark-grown seedlings to RS-inducing high light intensity (high light, 310 μmols m −2 s −1 ; Supplementary Fig. 23 ), compared with lower light levels (130 μmols m −2 s −1 , defined here as ‘low light’ for convenience). Under high light intensity, we detected GUN1-mediated repression of deetiolation within 3 h ( Fig. 5a,b ), consistent with the effect of lincomycin on early deetiolation responses to the dark-to-low light transition ( Fig. 1c ). Under these conditions, we observed that the rapid, low light induction of GLK1 expression was significantly reduced by high light intensity, whereas induction levels of GLK1 expression in gun1 were similar in low and high light ( Fig. 5c , Supplementary Fig. 24 ). This result suggests that high light intensities can antagonize the low-light induction of GLK1 expression, at least in part through GUN1-mediated RS. In agreement with this conclusion, analysis of the available data [35] indicates that high light intensities prevent the informational low-light induction of GLK1-induced genes, a behaviour that is similar for the genes in ‘Gene-Set PIF-RS’ or the genes whose light-induction is inhibited by RS ( Fig. 5d ). Because PIF3 levels in the WT and gun1 were below the level of detection in both low and high light ( Fig. 5e ), and pifq deetiolation and GLK1 induction was slower under high light than low light ( Supplementary Fig. 25 ), our findings collectively support the notion that GLK1 expression under high light is repressed in a PIF-independent fashion by a GUN1-facilitated pathway, to antagonize the light induction of the photomorphogenic programme. Moreover, in agreement with the role we propose for GLK1 as downstream effector of both informational-light and RS, we found that GLK1-OX seedlings were largely insensitive to high light intensity and underwent deetiolation similarly in both low and high light ( Fig. 5f ). On the basis of these assembled data, we conclude that activation of GUN1-mediated RS by high light during early deetiolation represses informational-light-induced derepression of GLK1 , attenuating hook unfolding and cotyledon separation. This might protect the seedling by minimizing the exposed cotyledon surface to avoid excess light damage, adding to other high light-induced strategies like excess light dissipation [33] , [36] . Consistent with this notion, survival of gun1 mutants during deetiolation under high light is significantly poorer than WT [13] , [37] . 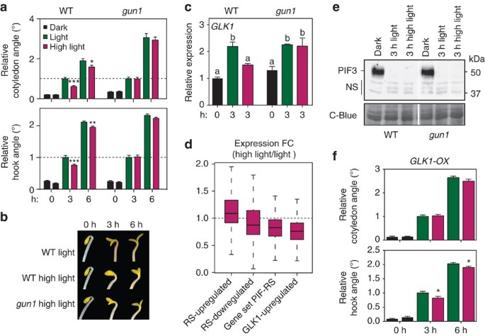Figure 5: High-intensity light induces GUN1-facilitated RS and inhibits PIF-mediated early light-induced deetiolation. (a) Hook unfolding and cotyledon separation were significantly slower in dark-grown WT seedlings after 3 and 6 h of high light treatment (purple) compared with light (green), whilegun1mutant seedlings were insensitive to high light and deetiolated at the same rate in both light and high light. Values for each genotype are expressed relative to the corresponding value in light at 3 h set at one (n⩾65). (b) Visual phenotype of representative seedlings ina. (c) Light-induction ofGLK1in dark-grown WT seedlings is significantly reduced in high light (purple) compared with light (green), whilegun1mutant seedlings are insensitive to high light and reached similar levels ofGLK1induction in light and high light. Data are the means±s.e.m. of biological triplicates (n=3). Different letters denote the statistically significant differences among means (Tukey-b test). (d) Fold-change expression between WT seedlings grown in high light and light for the following gene sets: RS-upregulated27, RS-downregulated27, Gene-Set PIF-RS and GLK1-upregulated17. Data were obtained from ref.35. (e) PIF3 protein levels in WT andgun1dark-grown seedlings were below level of detection after 3 h in light or in high light. (f)GLK1-OXseedlings were largely insensitive to high light and deetiolated similarly in both light (green) and high light (purple;n⩾45). Inaandf, error bars represent s.e.m. and the statistically significant differences between light treatments at each time point by Student’st-test are shown (*P<0.05; **P<0.01 and ***P<0.001). The experiments were repeated two times with similar results. C-blue, coomassie blue; NS, non-specific bands. Figure 5: High-intensity light induces GUN1-facilitated RS and inhibits PIF-mediated early light-induced deetiolation. ( a ) Hook unfolding and cotyledon separation were significantly slower in dark-grown WT seedlings after 3 and 6 h of high light treatment (purple) compared with light (green), while gun1 mutant seedlings were insensitive to high light and deetiolated at the same rate in both light and high light. Values for each genotype are expressed relative to the corresponding value in light at 3 h set at one ( n ⩾ 65). ( b ) Visual phenotype of representative seedlings in a . ( c ) Light-induction of GLK1 in dark-grown WT seedlings is significantly reduced in high light (purple) compared with light (green), while gun1 mutant seedlings are insensitive to high light and reached similar levels of GLK1 induction in light and high light. Data are the means±s.e.m. of biological triplicates ( n =3). Different letters denote the statistically significant differences among means (Tukey-b test). ( d ) Fold-change expression between WT seedlings grown in high light and light for the following gene sets: RS-upregulated [27] , RS-downregulated [27] , Gene-Set PIF-RS and GLK1-upregulated [17] . Data were obtained from ref. 35 . ( e ) PIF3 protein levels in WT and gun1 dark-grown seedlings were below level of detection after 3 h in light or in high light. ( f ) GLK1-OX seedlings were largely insensitive to high light and deetiolated similarly in both light (green) and high light (purple; n ⩾ 45). In a and f , error bars represent s.e.m. and the statistically significant differences between light treatments at each time point by Student’s t -test are shown (* P <0.05; ** P <0.01 and *** P <0.001). The experiments were repeated two times with similar results. C-blue, coomassie blue; NS, non-specific bands. Full size image Our findings support a mechanistic model ( Fig. 6 ), whereby the PIFs directly repress GLK1 expression in the dark to support skotomorphogenesis. In the light, phytochrome-induced degradation of the PIFs relieves the repression of GLK1 expression and this permits initiation of photomorphogenic development, as long as the plastid is functionally intact, through GLK1 regulation of photosynthetic genes [17] and potentially of as yet undefined genes involved in the regulation of other facets of photomorphogenesis (putative ‘Gene(s) X’ in Fig. 6 ). In conditions where the plastid is damaged, RS is activated and antagonizes the phytochrome-signal output by repressing the light-induced derepression of GLK1 , through a GUN1-facilitated, PIF-independent pathway, which effectively attenuates normal photomorphogenesis for the purpose of protecting the seedling. According to this model, whereas the phytochrome/PIF system monitors dark-light transitions, as well as light quality and periodicity, to optimize light-regulated development, the chloroplast functions as a sensor of excess light (at levels where the phytochrome/PIF system is saturated), to prevent potentially irreversible damage. Hence, coincidence of external light stimuli and internal chloroplast integrity is necessary to promote photomorphogenesis. 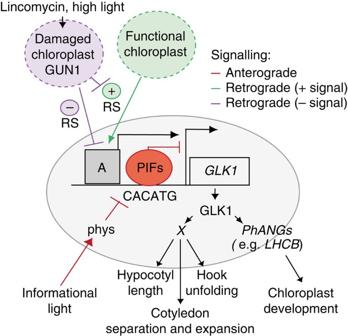Figure 6: Antagonistic actions of PIF-mediated light signalling and GUN1-mediated plastid RS in regulating photomorphogenesis. PIFs bind to theGLK1promoter through a PBE motif (CACATG)16to directly repressGLK1expression in the dark. Unknown transcriptional activator(s) represented by A sits on the promoter constitutively poised to activateGLK1expression. In response to the informational light signals, activated phytochromes induce degradation of the PIFs, triggering the derepression ofGLK1expression, driven by A. In turn,GLK1directly induces expression of photosynthesis-associated nuclear genes (PhANGs)17, and of one or more putative ‘Gene(s) X’ that implement other aspects of photomorphogenesis. If chloroplast integrity is disrupted by lincomycin or high light, a negative retrograde signal ((−) RS) emitted by dysfunctional chloroplasts induces GUN1-mediated repression ofGLK1expression by repressing the effectiveness of A. Alternatively, functionally intact chloroplasts might produce a positive RS ((+) RS) necessary for the expression and/or activity of A, that is disrupted in a GUN1-facilitated manner when chloroplast function is altered. Figure 6: Antagonistic actions of PIF-mediated light signalling and GUN1-mediated plastid RS in regulating photomorphogenesis. PIFs bind to the GLK1 promoter through a PBE motif (CACATG) [16] to directly repress GLK1 expression in the dark. Unknown transcriptional activator(s) represented by A sits on the promoter constitutively poised to activate GLK1 expression. In response to the informational light signals, activated phytochromes induce degradation of the PIFs, triggering the derepression of GLK1 expression, driven by A. In turn, GLK1 directly induces expression of photosynthesis-associated nuclear genes ( PhANGs ) [17] , and of one or more putative ‘ Gene(s) X ’ that implement other aspects of photomorphogenesis. If chloroplast integrity is disrupted by lincomycin or high light, a negative retrograde signal ((−) RS) emitted by dysfunctional chloroplasts induces GUN1-mediated repression of GLK1 expression by repressing the effectiveness of A. Alternatively, functionally intact chloroplasts might produce a positive RS ((+) RS) necessary for the expression and/or activity of A, that is disrupted in a GUN1-facilitated manner when chloroplast function is altered. Full size image Activation of RS has been proposed, alternately, to involve both positively and negatively acting configurations [30] , [38] . In principle, our data are consistent with either possibility, in which lincomycin would, respectively, either (a) disrupt a positive intact-plastid-emitted signal, which acts in a GUN1-regulated manner and is necessary for the expression of GKL1 following derepression by PIF removal, or (b) induce a negative plastid-emitted signal, which acts to repress the nuclear transcription of GLK1 in a GUN1-mediated manner ( Fig. 6 ). In either configuration, our observation that the cop -like phenotype of pifq is suppressed by lincomycin in the dark suggests that activation of RS by plastid malfunction is independent of light, consistent with previous reports of RS activity in darkness [19] , [27] . Although the mechanism by which RS repress light-induced derepression of GLK1 expression remains unknown, our results establish that the process requires GUN1, is independent of the PIFs, and does not appear to involve GUN5, GUN6 or ABI4 (in agreement with Kakizaki et al . [18] ), and might involve regulation at the transcriptional and/or post-transcriptional levels through a factor or factors (‘A’ in our model in Fig. 6 ) of yet unknown nature. Plant materials and growth conditions Arabidopsis thaliana seeds used in these studies have been described elsewhere, including pifq (ref. 10 ), glk1.1 (ref. 39 ) , GLK1-OX and GLK2-OX lines (ref. 40 ), abi4-t (ref. 41 ), gun5-1 (ref. 21 ), gun6-1D (ref. 30 ), cop1-4 (ref. 42 ) and hy5-215 (ref. 43 ), all in the Columbia (Col-0) ecotype, and sigma2-1 (ref. 44 ) and sigma6 (soldat8 ; ref. 45 ) in the WS and L er and ecotypes, respectively. The newly described gun1 allele ( gun1-201 ) corresponds to insertion line SAIL_290_D09 obtained from ABRC ( Supplementary Fig. 26 ). Seeds were sterilized and plated on medium without sucrose as described [46] . Seedlings were then stratified for 4 days at 4 °C in darkness, and then placed under continuous white light (1 μmol m −2 s −1 ), red light (1.3 μmol m −2 s −1 ) or darkness for 3 days, except in experiments shown in Fig. 1c , performed using a white light intensity of 25 μmol m −2 s −1 , and in Fig. 5 , performed using a combination of red (60%) and blue (40%) light, where Light corresponds to 130 μmol m −2 s −1 and High light to 310 μmol m −2 s −1 . Fluence rates were measured with a Spectrosense2 metre associated with a 4-channel sensor [47] . For lincomycin treatments, media was supplemented with 0.5 mM lincomycin (Sigma L6004) or as indicated ( Supplementary Fig. 4 ) [19] . For norflurazon treatment, media was supplemented with 5 uM norflurazon (Novartis 100–848-AA). To measure hypocotyl length, hook angle and cotyledon angle and area, seedlings were arranged horizontally on a plate and photographed using a digital camera (Nikon D80). Measurements were performed using NIH Image software (Image J, National Institutes of Health) [48] . At least 25 seedlings were measured to calculate the mean and s.e.m. in at least two biological replicates. In Supplementary Fig. 25 , the response to light was measured in individual pifq seedlings across time. Gene expression analysis Quantitative RT–PCR, RNA extraction, cDNA synthesis and qRT–PCR were done as described [48] . Briefly, 1 μg of total RNA extracted using the RNeasy Plant Mini Kit (Qiagen) were treated with DNase I (Ambion) according to the manufacturer’s instructions. First-strand cDNA synthesis was performed using the SuperScript III reverse transcriptase (Invitrogen) and oligo dT as a primer (dT30). cDNA was then treated with RNase Out (Invitrogen) before 1:20 dilution with water, and 2 μl was used for real-time PCR (Light Cycler 480; Roche) using SYBR Premix Ex Taq (Takara) and primers at a 300 nM concentration. Gene expression was measured in three independent biological replicates (with the exception of Supplementary Fig. 6b (one), Supplementary Fig. 23 (four) and Supplementary Figs 24 and 25 (two)), in at least three technical replicates for each biological sample. PP2A ( AT1G13320 ) was used for normalization [49] . Primers used to analyse LHCB1.4 ( AT2G34430 ) and LHCB2.2 ( AT2G05070 ) were described previously [10] , [27] . GLK1 ( AT2G20570 ) expression was measured using primers 5′- GCTACGAGATTTAGAGCACCG -3′ and 5′- TTGACGGATGTAAGTCTACCG -3′, and GUN1 ( AT2G31400 ) expression using primers 5′- TGAGTATATTGACTGGCTGGG -3′ and 5′- GCATTTTGACAGGTGGAATGG -3′. RNA-seq library construction and data processing Total RNA from 3-day-old dark-grown seedlings was extracted using QIAshredder columns and the RNeasy Plus Mini Kit (Qiagen). RNA-seq libraries were prepared using Illumina’s directional mRNA-seq sample preparation following the manufacturer’s protocol with some modifications. The mRNA was purified from 20 μg of total RNA using Dynabeads Oligo (dT) 25 (Invitrogen) and fragmented using Fragmentation Reagents (Ambion). The resulting polyA-tailed 3′-end fragments were captured using Dynabeads Oligo (dT) 25 (Invitrogen), and then treated by Antarctic Phosphatase (NEB) and T4 Polynucleotide Kinase (NEB). The sample was purified using RNeasy MinElute Cleanup Kit (Qiagen) and Illumina's SRA 5′-adaptor was ligated to the eluted mRNA fragments by T4 RNA Ligase 1 (NEB). Reverse transcription was performed using the SuperScript III First-Strand Synthesis System (Invitrogen) and the 3′-cDNA adaptor derived from Illumina’s v1.5 sRNA 3′-adaptor conjugated with the anchored oligo (dT) 20 primer. The first-strand cDNA was purified using the Agencourt AMPure XP system. The second-strand cDNA was synthesized and amplified by PCR using Phusion High-Fidelity DNA Polymerase with Illumina's sRNA PCR primer set. The library was purified using the Agencourt AMPure XP system and the size was validated by Bioanalyzer 2000 (ref. 50 ). Libraries from triplicate biological samples were sequenced on the Illumina HiSeq platform. Reads were aligned to the TAIR10 representative transcriptome using Bowtie [51] with one mismatch allowed. To prevent false counts, mapping was performed using the 3′-end 500-bp region of the coding strand. Differentially expressed genes were identified using the edgeR package [52] among those genes in which at least 2 of the 6 samples being compared had ⩾ 5 reads per million. SS genes were defined as those that differ with a P value≤0.05 (adjusted for false-discovery rate), and SSTF genes as those that differ by more than or equal to twofold with a P value≤0.01 (adjusted for false-discovery rate) [11] ( Supplementary Fig. 27 ). Microarray data comparison and transcript analysis Expression data shown in Figs 2b , 3c,d and 4c , and Supplementary Figs 8b, 11b and 18b , were obtained from microarray data from GSE5770 (ref. 23 ) and GSE17159 (ref. 11 ). As a control, gene expression in the shared WT Light sample from the two experiments were first compared in each subgroup of genes analysed in each figure to validate that there were no statistically significant differences and thus the rest of the samples were comparable. Represented WT light values in Figs 2b and 4c , and Supplementary Figs 8b, 11b and 18b , are from ref. 23 . Expression data shown in Fig. 5d were obtained from GSE7743 (ref. 35 ). Promoter analysis for DNA-binding motifs Analysis was performed using the ‘Motif Analysis’ tool available at The Arabidopsis Information Resource ( http://Arabidopsis.org/tools/bulk/motiffinder/index.jsp ) for statistically overrepresented 6-mer motifs in the 500-bp genomic sequence upstream of the start codon of genes in gene-set PIF-RS, the SCOPE motif finder ( http://genie.dartmouth.edu/scope/ ), and the Arabidopsis Gene Regulatory Information Server ‘Agris’ ( http://arabidopsis.med.ohio-state.edu/AtTFDB/ ). Statistics Gene expression and morphological data shown in Figs 1b , 4 and 5c , and Supplementary Figs 2, 5b, 6c, 7, 14b, 15b, 18a, 19a, 22b, 24 and 25b , were analysed by one-way analysis of variance, and the differences between means were evaluated using Tukey-b post hoc multiple comparison test (IBM SPSS Statistics Software). Statistically significant differences were defined as those with a P value<0.05. Morphological and expression data were analysed using Excel (Microsoft) for statistically significant differences from their control. P values were determined by homoscedastic Student’s t -test for data in Figs 1c , 4b,d and 5a,f , and Supplementary Figs 1b, 4, 6b, 20, 21, 22c, 25a and 26b , and WT and pifq in Fig. 1e , and by heteroscedastic Student’s t -test for data in Figs 2b , 3c and 4c , and Supplementary Figs 8b and 18b . Statistically significant differences were defined as those with a P value<0.05. In the figures significance level is indicated as * P <0.05, ** P <0.01 and *** P <0.001. Hypergeometric tests shown in Fig. 4a and Supplementary Fig. 17 were performed using R. Protein extraction and immunoblots Protein extracts were prepared from 2-day-old dark-grown WT and gun1 seedlings transferred to white light for the time and light intensities indicated in Fig. 5e . Tissue samples were collected and frozen in liquid nitrogen, and samples were manually ground under frozen conditions before resuspension in extraction buffer. Protein extraction was performed in boiling extraction buffer (100 mM MOPS (pH 7.6), 2% SDS, 10% glycerol, 4 mM EDTA, 2 g l −1 aprotinin, 3 g l −1 leupeptin, 1 g l −1 pepstatin and 2 mM PMSF). Total protein was quantified using a Protein DC kit (Bio-Rad), and β-mercaptoethanol was added just before loading [53] . Aliquots from each sample containing equal amounts of total protein (150 μg) were subjected to 7.5% SDS-PAGE gels. Proteins were then transferred to Immobilon-P membrane (Millipore), and immunodetection of endogenous PIF3 was performed as previously detailed [54] using a rabbit anti-PIF3 polyclonal antibody [55] (1:10,000 dilution) incubated with Hikari solution (Nacalai Tesque). Peroxidase-linked anti rabbit secondary antibody (1:5,000 dilution; Amersham Biosciences NA934) and a SuperSignal West Femto chemiluminescence kit (Pierce) were used for detection of luminescence using LAS-4000 Image imaging system (Fujifilm). The membrane was stained with Coomassie blue as a loading control. The uncropped scan of the western blot shown in Fig. 5e is provided in Supplementary Fig. 28 . Transmission electron microscopy Cotyledons from 3-day-old dark-grown seedlings were fixed and processed as described in ref. 11 , except that a Leica EM PACT2-RTS high-pressure freezing machine (Leica Microsystems, Vienna, Austria) was used for the high-pressure freezing method. Ultrathin sections were visualized in a Jeol JEM1010 electron microscope (JEOL Ltd, Akishima, Tokyo, Japan). Images were recorded with a SIS Mega View III CCD camera. Accession codes: RNA-seq data reported in this study have been deposited in the Gene Expression Omnibus database under the accession number GSE78969 . How to cite this article: Martín, G. et al . Phytochrome and retrograde signalling pathways converge to antagonistically regulate a light-induced transcriptional network. Nat. Commun. 7:11431 doi: 10.1038/ncomms11431 (2016).